Spin–orbital dynamics in a system of polar molecules Spin–orbit coupling in solids normally originates from the electron motion in the electric field of the crystal. It is key to understanding a variety of spin-transport and topological phenomena, such as Majorana fermions and recently discovered topological insulators. Implementing and controlling spin–orbit coupling is thus highly desirable and could open untapped opportunities for the exploration of unique quantum physics. Here we show that dipole–dipole interactions can produce an effective spin–orbit coupling in two-dimensional ultracold polar molecule gases. This spin–orbit coupling generates chiral excitations with a non-trivial Berry phase 2 π . These excitations, which we call chirons, resemble low-energy quasiparticles in bilayer graphene and emerge regardless of the quantum statistics and for arbitrary ratios of kinetic to interaction energies. Chirons manifest themselves in the dynamics of the spin density profile, spin currents and spin coherences, even for molecules pinned in a deep optical lattice and should be observable in current experiments. Polar molecules [1] , [2] , [3] , [4] , [5] , [6] present a flexible platform for the exploration of quantum magnetism in many-body systems due to their strong and long-range dipole–dipole interactions and their rich internal structure of rotational levels. A few isolated rotational levels of a molecule represent an effective spin degree of freedom. Net spin–spin couplings can directly be generated by dipolar interactions even in frozen molecule arrays. Recent experiments [7] , [8] with molecules pinned in a deep optical lattice have demonstrated dipolar spin-exchange coupling. The anisotropic dipole–dipole interaction can also couple the spin degrees of freedom to the orbital motion of the molecules. Signatures of this type of coupling have been recently reported experimentally in bosonic magnetic atoms [9] , [10] , and have been noted for their potential to generate topological phases [11] , [12] , [13] , [14] . All previously predicted phenomena were limited to zero-dimensional systems [15] or weakly interacting bosonic systems at zero temperature or were tailored to particular experimental set-ups [16] , [17] , [18] , [19] , [20] , requiring, for example, complicated dressing techniques [12] , [13] . Here we demonstrate that an effective spin–orbit coupling (SOC) is inherent in the excitations of any two-dimensional (2D) system of polar molecules with a pair of degenerate N =1 rotational levels. These excitations, which we call chirons, are characterized by a non-trivial Berry phase 2 π . The same Berry phase is responsible for, for example, an unconventional quantum Hall effect in bilayer graphene [21] , [22] . Remarkably, in our system, SOC emerges due to interactions rather than being a single-particle effect, which adds significant richness to the physics and removes the fundamental limitations imposed by spontaneous emission present when single-particle SOC is artificially generated by light [11] , [23] , [24] , [25] , [26] . We present ways to detect chirality and Berry phase, for instance, by exciting rotational degrees of freedom in a finite spatial region. Generically, this leads to two fronts of spin and density currents, corresponding to the two branches of the chiron spectrum. The Berry phase 2 π manifests itself in the d- wave symmetry ∝ cos(2 φ ) of the spin projection onto the plane, where φ is defined in Fig. 1a . In addition, the SOC leads to population transfer between the excited rotational levels together with the formation of a vortex structure in the spatial density profile. We discuss the experimental conditions necessary for the observation of the described phenomena and provide numerical examples germane to current polar molecule experiments in which molecules are pinned in a deep optical lattice with sparse filling. 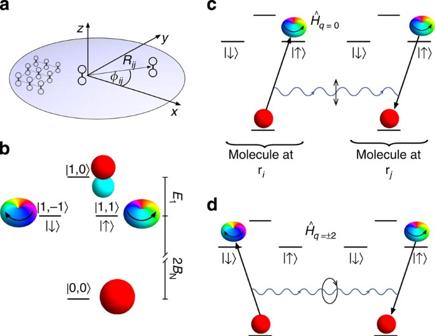Figure 1: The set-up. (a) Geometry: molecules confined in thexyplane, perpendicular to the quantization axisz; (Rij;φij) are the polar coordinates of the vectorRijjoining moleculesiandj. (b) Rotational levels of a molecule. The small icons mimic the angular distributions of the rotational states and are coloured according to their phase, the arrows showing the direction of the phase winding in the |1, ±1› states. (c,d) Processes involving dipolar exchange interactions. Inc, molecules exchange rotational levels while preserving both their total internal angular momentum and itsz-component. Ind, the internal angular momentum decreases by 2, while the orbital momentum of the two molecules increases by 2. Figure 1: The set-up. ( a ) Geometry: molecules confined in the xy plane, perpendicular to the quantization axis z ; ( R ij ; φ ij ) are the polar coordinates of the vector R ij joining molecules i and j . ( b ) Rotational levels of a molecule. The small icons mimic the angular distributions of the rotational states and are coloured according to their phase, the arrows showing the direction of the phase winding in the |1, ±1› states. ( c , d ) Processes involving dipolar exchange interactions. In c , molecules exchange rotational levels while preserving both their total internal angular momentum and its z -component. In d , the internal angular momentum decreases by 2, while the orbital momentum of the two molecules increases by 2. Full size image Many-body Hamiltonian for polar molecules in two dimensions We consider an ensemble of polar molecules confined in a plane perpendicular to an external electromagnetic field that sets the quantization axis z ( Fig. 1a ). The rotational spectrum of each molecule can be indexed by the rotational angular momentum N and its projection M onto the z axis ( Fig. 1b ). Throughout the paper, we set ħ = k B =1 and measure all lengths in units of the lattice constant a , unless specified otherwise. We assume that most molecules are in the ground rotational state ( N =0), and only the lowest-energy states, those with N =0 and N =1, participate in the dynamics. The N =1 states are separated from N =0 by a large gap 2 B N (~GHz), which significantly exceeds the characteristic interaction energy E d (~kHz). In addition, the |1, 0› state is separated from the |1, ±1› states by an energy scale E 1 , E d ≪ E 1 ≪ B N , for example, due to the presence of external electric field E ; more details on realising such level structure will be given below. Large lifetimes of the N =1 states ( ≳ 10 s) allow us to neglect relaxation between the N =1 and N =0 manifolds. The Hamiltonian for the system of polar molecules can be written as where the sums run over all particles in the system and is the single-particle Hamiltonian. Here, m is the mass of a molecule, U ( r ) is the external periodic potential and is the Hamiltonian of the internal degrees of freedom giving the spectrum in Fig. 1b . The dipole–dipole interaction between two molecules i and j with dipole moments and and separated by vector R ij ( Fig. 1a ) is given by Introducing polar coordinates R ij =( R ij , φ ij ), the interaction Hamiltonian (2) can be decomposed as where are spherical components of the dipole operator of molecule j . The operator , equation (4), conserves both the total internal angular momentum of the interacting molecule and its z -component. As shown in Fig. 1c , exchanges the states |1, ±1› and |0, 0› of two molecules while preserving M i + M j . Such ‘spin-exchange’ dipolar interactions have been observed in recent experiments on polar molecules [7] , Rydberg atoms [27] , [28] and magnetic atoms [29] . In contrast, the operator transfers angular momentum between the internal and external orbital motion of the molecules, while preserving the total projection onto the z axis. Namely, the operator decreases the internal angular momentum by 2, while increases the orbital angular momentum of a molecule by 2, thus preserving the total angular momentum (see, Fig. 1d ). As we shall show, this transfer of angular momentum is responsible for the generation of the effective SOC of the elementary excitations. Phenomenological analysis Let us assume that almost all the molecules are initially in their lowest rotational level |0, 0› and are in a spatially uniform, not necessarily equilibrium state, but with a relaxation time sufficiently long to be considered stationary. We then suppose that this state is slightly perturbed by a resonant microwave pulse, which excites a small number of molecules from |0, 0› to |1, ±1›. In what follows we show that the density and angular momentum dynamics of the |1, ±1› rotational levels after such excitation is equivalent to that of an ideal gas of spin-1/2 chiral quasiparticles (chirons). The emergence of the excitations can be phenomenologically understood as follows. Due to the translational invariance of the Hamiltonian of the system, the (quasi)momentum k (in the presence of an optical lattice), with polar coordinates ( k , φ k ) ( Fig. 2a ) is a good quantum number. In the long-wave limit k →0, there is a degeneracy between the excitations carrying molecules in the rotational states |↑›≡|1, 1› and |↓›≡|1, −1› due to the symmetry with respect to inverting the dipole moment. Note that the other excited rotational states are separated from |↑› and |↓› by large energy gaps and do not participate in the dynamics. This allows us to consider a reduced space {|↑›, |↓›} of rotational states. Each of these states can be obtained from the other by acting with the operators . 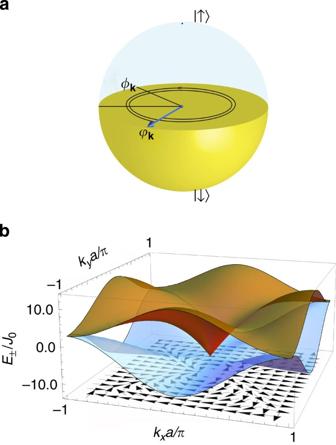Figure 2: Chiron states. (a) Chiron state on the Bloch sphere. (b) Chiron dispersion in a deep optical lattice in the first Brillouin zone forJ2=3J0. The lower (upper) surface corresponds toE+(k) [E_(k)]. The base of the plot shows the orientation of theE+branch Bloch vector in the equatorial plane. Hence, the most general form of the excitation Hamiltonian in the reduced space reads Figure 2: Chiron states. ( a ) Chiron state on the Bloch sphere. ( b ) Chiron dispersion in a deep optical lattice in the first Brillouin zone for J 2 =3 J 0 . The lower (upper) surface corresponds to E + ( k ) [ E _( k )]. The base of the plot shows the orientation of the E + branch Bloch vector in the equatorial plane. Full size image where k ± = k x ± ik y , and α ( k ) and ξ k are some functions of k . The Hamiltonian in equation (6) describes quasiparticles with a two-branch spectrum with energies corresponding to the eigenstates respectively, and a Berry phase of 2 π . In a system with an inversion-symmetric Hamiltonian, ĥ ( k )= ĥ (− k ), the Berry phase can be defined [30] modulo 4 π as an integral along a contour C connecting two points k and − k in momentum space. Thus, the Berry phase 2 π of chirons is non-trivial. As is necessary in a system with time-reversal symmetry [31] , [32] , Φ BP is a multiple of π . Let us notice that if α ( k )=const, the Hamiltonian (6) coincides with that of the low-energy excitations in bilayer graphene [21] , [22] in the wavelength limit k →0. In the next section, we demonstrate that such Hamiltonian is indeed realised in the case of weak interactions between the molecules. Microscopic calculation of the Hamiltonian In the previous section, we have shown phenomenologically that the effective Hamiltonian of long-wave excitations in a system of polar molecules has the form given by equation (6). In what immediately follows, we demonstrate that the Hamiltonian can be explicitly evaluated microscopically in the two opposite limits: when the kinetic energy is negligible compared with the characteristic interaction strength and when the interactions are small compared with the kinetic energy. While the first regime can be achieved by pinning the molecules in a deep optical lattice and is thus relevant for current experiments with reactive molecules [7] , the second regime could be in principle realised in the future with molecules that are non-reactive and less susceptible to überresonant processes [33] . To address the first limit, we consider molecules in a deep, unit-filled square optical lattice. In this setting, the translational degrees of freedom are frozen and dynamics occurs only in the internal degrees of freedom. The dynamics can be mapped to that of a gas of bosons with spin σ ε{↑,↓} and long-range hopping. The vacuum corresponds to all molecules being in the |0, 0› state. The effective Hamiltonian describing the rotational excitations can be expressed in terms of the bosonic creation and annihilation operators of rotational excitations with σ character at lattice site i ={ i x , i y }, as Here, the hopping constants J 0 and J 2 are determined by dipole matrix elements. We work in the hard-core limit, which restricts the occupation number on each site to 0 or 1. The hard-core constraint encapsulates that there is at most one molecule per lattice site and each molecule can harbour at most one N =1 rotational excitation. Physically, the hard-core constraint can stem either from strong elastic interactions or rapid inelastic loss rates, for example, two-body chemical losses, at short range [7] , [34] . The dispersions of a single rotational excitation are given by and shown in Fig. 2 . Here, F ( n ) ( k )=∑ j ≠0 exp(− i k · r j + inφ j )| r j | −3 with r j a vector connecting sites in the square lattice and φ j the polar angle of r j . The phase ϕ k of F (2) , that is, , determines the polar angle of the Bloch vector ( Fig. 2a ). In the long-wave limit, k →0, we obtain in accordance with equation (6) that ϕ k ≈2 φ k , ξ k / J 0 ≈ A +2 π / k and α ( k )=2 πJ 2 /(3 k ), with A ≈9.03. For general ratios J 2 / J 0 , both branches have a conical dispersion for small k . For the case J 2 =3 J 0 , as results from the geometry in Fig. 1a , there is a cancellation of the linear k component in the E + branch. This leads to a locally flat dispersion E + ( k )/ J 0 ≈ A +( k 2 ) and a conical dispersion E − ( k )/ J 0 ≈ A +4 πk +( k 2 ) ( Fig. 2b ). In the case of a sufficiently shallow optical lattice or weak interactions, the kinetic energy of the molecules can dominate over the mean interaction energy. In this case, the dynamics can be analysed perturbatively in the interactions. By explicitly evaluating the Hamiltonian of the excitations, the details of which are provided in Supplementary Methods , we reproduce equation (6) with the off-diagonal entry where the upper and the lower signs apply to bosonic and fermionic molecules, respectively; f 00 ( q ) is the distribution function of the molecules in the |0, 0› state. It is assumed to be stationary and independent of the molecule position, but it is not restricted to be in thermal equilibrium; q + = q x + iq y ; and ∫ q …=∫(2 π ) −2 … d 2 q . Due to the smallness of the interactions, the diagonal elements of the matrix in equation (6) are close to the kinetic energy of a single molecule and are only slightly modified by the interactions, ξ k ≈ k 2 (2 m ) −1 [1+(| d | 2 )]. This calculation is performed explicitly in Supplementary Methods . The long-time dynamics is dominated by small momenta. For an isotropic distribution function f 00 ( q )= f 00 ( q ), from equation (11) we find the value of the spin–orbital coupling in the limit k →0 to be For a Fermi liquid of fermionic molecules at zero temperature [ f 00 ( q )= θ ( k F − q )], equation (12) yields where k F is the Fermi momentum. At sufficiently high temperatures T ≫ n / m , where n is the density of the molecules (per nuclear spin), the distribution function is close to that of a Boltzmann gas, , and For cold atoms in a quadratic trapping potential, the density of the molecules depends on temperature as n ( T ) ∝ T −1 , resulting in the temperature dependency of the SOC α ( T ) ∝ T −3/2 . Chirality manifestations in spin and density dynamics The chirality of the excitations can be observed in the dynamics of the spin-1/2 operator, S ={ Ŝ x , Ŝ y , Ŝ z }, in the reduced space of the rotational levels |↑› and |↓›. Let us assume that a short laser pulse excites a group of molecules in a small region of characteristic size Λ around r =0, |0, 0›→|↑› (the results of this paper can be easily generalized to include more general excitation protocols, |0, 0›→ A ↑ |↑›+ A ↓ |↓›). The internal state |↑› corresponds to excitation by light with right-circular polarization x + iy , and has a definite phase winding, as shown in Fig. 1b . Hence, for a spatially isotropic distribution of excitations, the laser polarization is what determines the spatial phase pattern emerging during the dynamics. For sufficiently small Λ chirons leave the excited region quickly, reaching sufficiently low density, so that interactions between them can be neglected, and their dynamics is described by the kinetic equation for free particles, see Methods. In principle, chiron–chiron interactions may be important for hard-core particles in a deep optical lattice in the beginning of the dynamics, which, however, will not affect the results qualitatively. In the limit of pinned molecules, we additionally check whether chiron–chiron interactions can be neglected by numerically simulating the dynamics of two excitations, see Supplementary Methods and Supplementary Figs 2 and 3 . The chiral nature of the excitations is clearly visible in the density of Ŝ x where f ↑↑ ( r , q ) is the distribution function of the molecules in the | r , q › state at time t =0, v ± ( q ) are the velocities of the two chiron branches and φ q is the polar angle of the vector q . In the long-wave limit (see equation (7)) Equation (15) describes the spin distribution at sufficiently long times, when it is dominated by long-wave chirons ( q ≪ a −1 ). In this limit, the phase factor cos(2 φ q ) originates from the off-diagonal element of equation (6). To account for arbitrary-momenta excitations, 2 φ q in equation (15) has to be replaced by the polar angle ϕ q of a chiron state on the Bloch sphere ( Fig. 2a ). For the small Λ under consideration, the distribution has a d -wave symmetry at long times ( Fig. 3a,b ), which is a manifestation of the non-trivial Berry phase 2 π of the excitations. The radial distribution of the spin component after applying a narrow laser pulse depends on the molecular statistics, interaction strength, optical lattice depth and so on, while its d -wave symmetry is universal, being a consequence of the Berry phase 2 π . 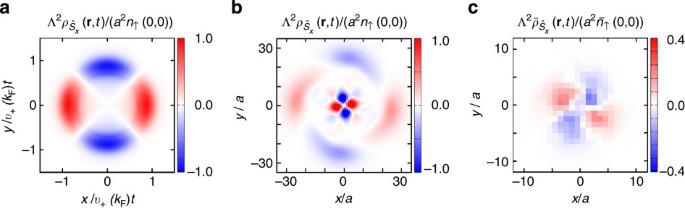Figure 3: Chiron spin dynamics. Spatial distributions of the spin coherences in a gas of polar molecules after applying a focused resonant pulse. (a) Density profile ofŜxin a weakly interacting Fermi liquid. (b) Density profile ofŜxin a deep optical lattice. (c) The density ofŜx, analogous tobbut for a lattice of 10% filling, averaged over disorder realizations (overbar denotes disorder average). The peak magnitude ofis reduced by a factor of ~20 compared with unit filling, but the symmetry is the same. Figure 3: Chiron spin dynamics. Spatial distributions of the spin coherences in a gas of polar molecules after applying a focused resonant pulse. ( a ) Density profile of Ŝ x in a weakly interacting Fermi liquid. ( b ) Density profile of Ŝ x in a deep optical lattice. ( c ) The density of Ŝ x , analogous to b but for a lattice of 10% filling, averaged over disorder realizations (overbar denotes disorder average). The peak magnitude of is reduced by a factor of ~20 compared with unit filling, but the symmetry is the same. Full size image The spatial distribution of the spin coherences can be particularly easily understood in the case of a Fermi liquid (fermionic molecules at low temperatures) with weak interactions. In this case, the excitations propagate at the maximal speed υ + ( k F ), k F being the Fermi momentum. At a distance r away from the initial excitation pulse, the spin distribution remains unaltered until time t = r / υ + ( k F ) when it is reached by the quickest branch of chirons with the angular distribution of spins . At a slightly later moment of time t = r / υ − ( k F ), the same point is reached by a wave of slower chirons with opposite spin, after which the spin density remains very small. The resulting distribution is shown in Fig. 3a . In the case of a deep optical lattice, the branch of chirons with the dispersion E − ( q ) is significantly faster than the other branch, leading to a quick spatial separation of the two branches ( Fig. 3b ) after applying the laser pulse. The outer circular density front corresponds to the faster chirons, which propagate at a nearly constant speed, while the more complex inner pattern comes from the slower branch of chirons. Despite different dispersions of the chirons, the angular distribution of the spin is again ∝ cos(2 φ ). Because of the SOC, spin is not conserved and the total numbers of molecules in the rotational states |↑› and |↓›, are time dependent. At long times t →∞, both N ↑ ( t ) and N ↓ ( t ) saturate at a half of the number N ex of the initially excited molecules ( Fig. 4c ) regardless of the details of the distribution function f ↑↑ ( r , q ). The total number of molecules in excited rotational states is conserved, N ↑ ( t )+ N ↓ ( t )= N ex . 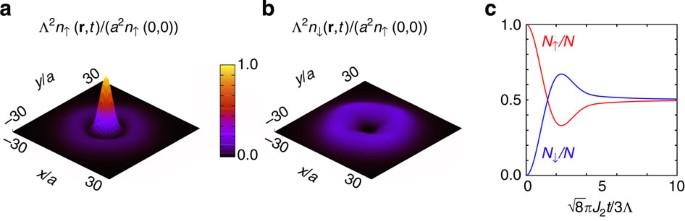Figure 4: Chiron density dynamics. Densities of |↑› (a) and |↓› (b). The vortex structure is clearly visible in the |↓› density. The density dipn↓(r,t)∝r4in the centre of the vortex structure is a manifestation of the Berry phase 2π. (c) Dynamics of the total spin populations in a deep optical lattice. The population of the two spin components undergoes a single oscillation before monotonically approaching 1/2. Figure 4: Chiron density dynamics. Densities of |↑› ( a ) and |↓› ( b ). The vortex structure is clearly visible in the |↓› density. The density dip n ↓ ( r , t ) ∝ r 4 in the centre of the vortex structure is a manifestation of the Berry phase 2 π . ( c ) Dynamics of the total spin populations in a deep optical lattice. The population of the two spin components undergoes a single oscillation before monotonically approaching 1/2. Full size image Thus, the SOC transfers the internal angular momentum of the molecules, all of which are in the |↑› state at t =0, to their orbital motion, leading to the formation of a vortex structure around r =0. This manifests itself, for instance, in a dip in the density of molecules in the |↓› rotational state, , around the centre of the vortex structure ( Fig. 4b ). In particular, if the chiron spectrum has a branch with quadratic dispersion E ( k )~ k 2 (2 M ) −1 , which is realised, for example, for weak interactions in a shallow optical lattice or for strong interactions in a deep optical lattice, the density of the spin-down molecules close to the centre of the vortex estimates n ↓ ( r , t )~( M 2 r 2 / t 2 ) 2 N ex /Λ 2 at sufficiently long times. Far from the centre of the vortex, the density profile is described by freely propagating chirons that do not interfere with each other: The two contributions in the sum in equation (19) correspond to the two branches of chirons propagating with velocities υ + ( q ) and υ − ( q ), which leads to their spatial separation. Experimental accessibility In this section, we discuss some details related to the observation of dipolar SOC in present cold polar molecule experiments, taking as a representative example the KRb experiment at JILA [7] . To prevent chemical reactions, KRb polar molecules are pinned in a deep 3D optical lattice. The relevant energy scales for equation (9) are and J 2 =3 J 0 . Trapping in a deep optical lattice may also be required for molecular species that are chemically stable, as the presence of a very high density of resonances at ultracold energies has been proposed to lead to long-lived collision complexes, which are highly susceptible to three-body loss [33] . The chirons’ spectra in the entire Brillouin zone can be measured by means of Rabi spectroscopy provided the probe beam can transfer the required quasi-momentum k R ≃ 1/ a to the molecules. Direct microwave transitions are insufficient since they have k R a ≪ 1, but k R a ≃ 1 can be achieved using optical Raman pulses. Here, k R =| k 1 − k 2 |, with k i the wavevector of the i th Raman beam. Raman transitions between internal states are already a key part of the production of ground-state molecules through STIRAP [35] ; our proposal requires only minor modifications of this well-established procedure. Due to the inherent difficulty of directly cooling molecules, present experiments are not quantum degenerate, leading to a sparse lattice-filling fraction near 10% [7] , [8] , [34] . Figure 3c displays the density of Ŝ x in a lattice with 10% filling, averaged over disorder realizations. The d -wave symmetry of the distribution is still visible, albeit with reduced contrast compared with the unit-filled case ( Fig. 3b ). The d -wave symmetry is a consequence of the Berry phase, a topological property, and so is robust against disorder. In contrast, disorder smears the vortex structure. In the rotational structure of KRb, nuclear quadrupole interactions cause the states with predominant |1, −1› and |1, 1› character to be non-degenerate by about 70 h kHz at the 545 G magnetic fields used for magneto-association [36] . These states can be made degenerate and out of resonance with the |1, 0› level by increasing the strength of the magnetic field B , even at zero electric field. In this scenario, the B field determines the quantization axis. For 40 K 87 Rb, where the nuclear quadrupole moments are ( eqQ ) Rb =−1.380 h MHz and ( eqQ ) K =0.452 h MHz [36] , the levels cross near B ≃ 1,260 G, well within experimental feasibility. The energy difference between these levels close to the crossing is nearly linear, with a slope of roughly 40 Hz G −1 . Stabilization of magnetic fields at the 10 mG level, which is routine in ultracold gas experiments, would correspond to non-degeneracy on the order of 0.4 Hz, and will not significantly affect our results. Similar comments apply for the other alkali metal dimers. The level structure in Fig. 1b also results for 1 Σ molecules without hyperfine structure, for example, bosonic SrO, in the presence of a uniform electric field. Finally, we note that several knobs can be used to manipulate the Hamiltonian, equation (9). For example, by changing the angle of the quantization axis with respect to the space-fixed z axis, one can tune the ratio J 2 / J 0 and remove the cancellation seen in the E + branch. This can be used in turn to control the propagation velocity of the two branches of chirons. Chiron–chiron interactions that fall off as 1/ r 3 can also be controllably introduced by turning on an external static electric field. We have demonstrated that a 2D system of polar molecules behaves as a gas of chiral excitations with a Berry phase 2 π . We have shown that signatures of those excitations, which resemble the low-energy excitations exhibited by bilayer graphene, manifest in both the dynamics of the density and spin coherences. The implementation of SOC in polar molecules presented here can open other exciting research avenues. In particular, by superimposing an effective magnetic field to the chirons via light-generated synthetic gauge fields [23] , it might be possible to simulate the unconventional quantum Hall effect of bilayer graphene and to see its intriguing consequences [21] in the lowest Landau levels in the limit of low chiron density and high synthetic magnetic fields. Such an effect would require fermionic statistics of the excitations, which can be realised with fermionic molecules in a shallow optical lattice. Although so far the system in consideration is an ideal or nearly ideal gas of chirons and interactions between them can be neglected, chiron–chiron interactions tunable by the duration of the laser pulse, the size of the excited region or an external electric field may lead to very rich physics. For example, chiron–chiron interactions together with non-stationary background N =0 molecules or microwave dressing can give rise to interesting dynamic structures, new types of transport phenomena and even to fractional quantum Hall phases when combined with synthetic gauge fields [13] , [37] . Finally, we expect our predictions to be extendable to other dipole–dipole interacting systems such as Rydberg atoms, magnetic atoms and magnetic defects in solids. Kinetic equation for polar molecules To characterize the dynamics of a system of polar molecules, we introduce the non-equilibrium Green’s functions where σ and σ ′ label the internal states of the molecules ( σ corresponds to (|1, −1›, |0, 0›, |1, 1›)). The upper (lower) sign applies to bosonic (fermionic) particles. The distribution functions of the molecules are defined as where the upper and the lower signs apply to bosonic and fermionic particles, respectively, and is the result of the Wigner transformation [38] , [39] of . Using the functions (20) and (21), we define a 2 × 2 matrix in the Keldysh space [38] , [39] , Each of the Green’s functions in equation (23) is a matrix in the space of the internal rotational levels of the molecules. The function (23) satisfies the equation (Dyson equation minus its conjugate), where ; 1=( t 1 , r 1 ), 2=( t 2 , r 2 ) and is the self-energy part, determined by the dipole–dipole interactions. In terms of the distribution functions , the kinetic equation reads where U ( r ) is the external smooth (trapping) potential, E p is the kinetic (quasi)energy, the summation over repeated indices is implied, and St f is the collision integral, which accounts for the relaxation of the distribution function due to molecular collisions. In this paper, we consider a model with a small relaxation rate, which can be neglected on the characteristic times of interest, so that the excitations propagate ballistically. Also, we assume that chirons reach sufficiently low density shortly after they are excited, so that chiron–chiron interactions can be neglected, and the problem becomes effectively single particle. Introducing the chiron annihilation operator where are the annihilation operators for the plane-wave states in the reduced space {|↓›, |↑›} of the rotational levels of the molecules and the kinetic equation (25) is reduced, under the assumptions made above, to that for a single-particle problem with the dispersion E ± ( k ): In the case U =0, considered in this paper, the most general solution of equation (27) reads G ± ( r , p ) being arbitrary functions of two arguments. How to cite this article : Syzranov, S. V. et al. Spin–orbital dynamics in a system of polar molecules. Nat. Commun. 5:5391 doi: 10.1038/ncomms6391 (2014).